RUNX1-induced silencing of non-muscle myosin heavy chain IIB contributes to megakaryocyte polyploidization Megakaryocytes are unique mammalian cells that undergo polyploidization (endomitosis) during differentiation, leading to an increase in cell size and protein production that precedes platelet production. Recent evidence demonstrates that endomitosis is a consequence of a late failure in cytokinesis associated with a contractile ring defect. Here we show that the non-muscle myosin IIB heavy chain (MYH10) is expressed in immature megakaryocytes and specifically localizes in the contractile ring. MYH10 downmodulation by short hairpin RNA increases polyploidization by inhibiting the return of 4N cells to 2N, but other regulators, such as of the G1/S transition, might regulate further polyploidization of the 4N cells. Conversely, re-expression of MYH10 in the megakaryocytes prevents polyploidization and the transition of 2N to 4N cells. During polyploidization, MYH10 expression is repressed by the major megakaryocyte transcription factor RUNX1. Thus, RUNX1-mediated silencing of MYH10 is required for the switch from mitosis to endomitosis, linking polyploidization with megakaryocyte differentiation. Platelets, the blood cells involved in haemostasis, arise in mammals from the fragmentation of the cytoplasm of a giant cell called megakaryocyte (MK) [1] , [2] . The large cell size is related to polyploidization, a unique process that is an integral part of MK differentiation [3] . The process of polyploidization, which is denoted as endomitosis [4] , corresponds to repeated incomplete cell cycles marked by abortive mitosis at the late phase of cytokinesis [5] , [6] and generates cells with ploidy of 2N x with a modal ploidy of 16N [3] , [4] . In contrast to other cells undergoing failure of cytokinesis, MK contain a single polylobulated nucleus. At the 2N to 4N transition, cleavage furrow ingression occurs, but subsequently regresses with a backward movement between the two daughter cells [5] , [6] . A similar phenomenon is observed at higher ploidy with a less profound furrow ingression [7] , [8] . The cleavage furrow is related to the development at the equator of a contractile ring consisting of myosin II and F-actin, an actomyosin complex generating the forces necessary for furrow ingression and cell separation [9] . Our previous results have shown that there was a very limited accumulation of non-muscle myosin IIA (MYH9) in the contractile ring of MK undergoing mitosis or endomitosis, but the existence of furrow ingression suggested that a myosin II activity still persisted in endomitosis [6] . In this study, we investigated the presence of MYH10 and showed that it is expressed in immature MK where it accumulates in the contractile ring, and that its expression is silenced during differentiation. MYH10 downregulation increases the ploidy level, and inversely, MYH10 overexpression decreases the ploidy level. Moreover, we show that the Runt related transcription factor 1 (RUNX1) negatively regulates MYH10 expression and thus links the polyploidization process with terminal MK differentiation. MYH9 does not have an important role in MK endomitosis First, we confirmed an almost complete absence of MYH9 accumulation in the contractile ring during MK mitosis or endomitosis ( Fig. 1a ) opposite to primary erythroblasts undergoing mitosis ( Fig. 1b ). MYH9 has been considered as the only non-muscle myosin II heavy chain expressed in MK and platelets [10] . Therefore, we studied MK-restricted myh9 knock-out (KO) mice ( myh9 f/f(PF4 Cre+) ) to examine the role of MYH9 in MK ploidization [11] , [12] , expecting an increase in MK ploidy. Surprisingly, no significant difference in the in-vivo MK ploidy level between myh9 f/f(PF4 Cre+) (17.11N, n =6) and control mice ( myh9 f/f(PF4 Cre-) ; 16.53N, n =4, P =0.22, t -test, ploidy measured in MK≥8N) was seen ( Fig. 1c ). Blebbistatin, a small molecule inhibitor of myosin [13] , [14] , has been recently shown to increase MK ploidy [15] . Addition of 50 μM blebbistatin (an enantiomer mixture) [16] in culture led to an increase in MK mean ploidy level that was similar between myh9 f/f(PF4 Cre+) and control mice (from 10.40N to 14.72N, P= 0.01, t -test, for myh9 f/f(PF4 Cre+) mice, and from 10.00N to 13.40N, P =0.01, t -test, for control mice, n =3, ploidy measured in MK≥8N; Fig. 1d ). 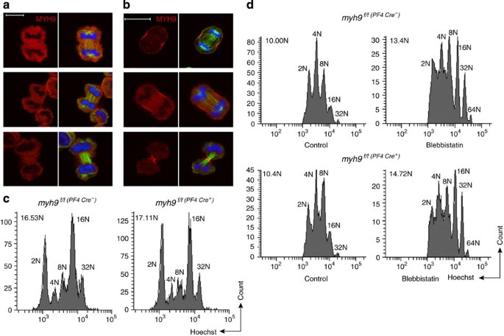Figure 1: Blebbistatin increased ploidy ofmyh9KO MK. (a,b) Human MKs were derived from CD34+cells and were studied at day 8 of culture. Cells were deposited on polylysine-coated slides, fixed and stained for tubulin (α and β, green) and MYH9 (red). DNA was stained with TOTO (blue). The accumulation of MYH9 in the contractile ring was compared between MK undergoing mitosis or endomitosis (a) and primary mitotic erythroblasts (b). Scale bars represent 10 μm. (c) The ploidy of murine MK was studied after double staining with an anti-CD41 antibody and Hoechst labelling. The histograms show the ploidy level (≥8N) of bone marrow MK frommyh9f/f (PF4 Cre+)(17.11N,n=6) and controlmyh9f/f (PF4 Cre−)mice (16.53N,n=4). (d) Ploidy levels of MK (≥8N) derived from the fetal liver ofmyh9f/f (PF4 Cre+)and control mice and treated with myosin II inhibitor blebbistatin (50 μM in DMSO) or without (DMSO). The increase in mean ploidy induced by blebbistatin was similar formyh9f/f (PF4 Cre+)mice (10.40N–14.72N;P=0.01,t-test;n=3) and control mice (10.00N–13.40N;n=3,P=0.01,t-test). Figure 1: Blebbistatin increased ploidy of myh9 KO MK. ( a , b ) Human MKs were derived from CD34 + cells and were studied at day 8 of culture. Cells were deposited on polylysine-coated slides, fixed and stained for tubulin (α and β, green) and MYH9 (red). DNA was stained with TOTO (blue). The accumulation of MYH9 in the contractile ring was compared between MK undergoing mitosis or endomitosis ( a ) and primary mitotic erythroblasts ( b ). Scale bars represent 10 μm. ( c ) The ploidy of murine MK was studied after double staining with an anti-CD41 antibody and Hoechst labelling. The histograms show the ploidy level (≥8N) of bone marrow MK from myh9 f/f (PF4 Cre+) (17.11N, n =6) and control myh9 f/f (PF4 Cre−) mice (16.53N, n =4). ( d ) Ploidy levels of MK (≥8N) derived from the fetal liver of myh9 f/f (PF4 Cre+) and control mice and treated with myosin II inhibitor blebbistatin (50 μM in DMSO) or without (DMSO). The increase in mean ploidy induced by blebbistatin was similar for myh9 f/f (PF4 Cre+) mice (10.40N–14.72N; P =0.01, t-test ; n =3) and control mice (10.00N–13.40N; n =3, P =0.01, t -test). Full size image MYH10 is expressed in the contractile ring of MK As blebbistatin inhibits all myosin II isoforms [14] , we investigated the expression of the three non-muscle isoforms MYH9, MYH10 and MYH14 during human and mouse MK differentiation. We differentiated hematopoietic progenitors (CD34 + cells for human and lineage-negative cells for mouse) in the presence of thrombopoietin (TPO), the growth factor regulating MK development [2] . The MKs were sorted by platelet-specific membrane glycoprotein CD41 (CD41 + ). MYH14 was undetectable during MK differentiation, whereas MYH10 messenger RNA (mRNA) and protein were identified by quantitative reverse transcription (RT)–PCR and western blot analyses in undifferentiated MK. During human MK differentiation, MYH10 expression markedly decreased from day 6 to day 9, approximately at a time when MK have switched from mitosis to endomitosis, to become undetectable in mature MK (day 12) and blood platelets, whereas MYH9 expression increased ( Fig. 2a and b ). This inverse link between MYH10 expression and differentiation was confirmed by directly sorting cord blood CD34 + -derived MK on the CD41 and CD42 expression at day 10 of culture. An important decrease in MYH10 expression, and inversely, an increase in MYH9 expression were detected at the protein and mRNA level in CD41 high CD42 high MK in comparison with CD34 + CD41 − cells and immature MK (CD41 low CD42 low ; Fig. 2c and d ). During murine MK differentiation, MYH9 expression remained stable, whereas MYH10 expression was hardly detectable as soon as 24 h after the beginning of the culture ( Fig. 2e and f ). 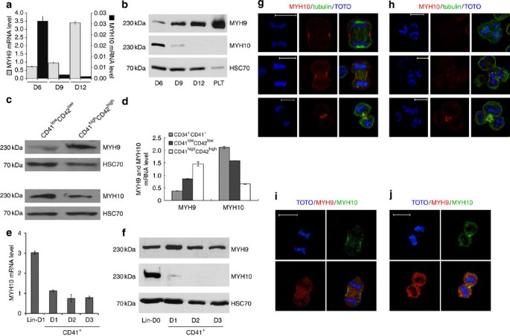Figure 2: MYH10 is expressed during MK differentiation. (a,b) CD41+MKs were derived from adult blood CD34+cells and studied at three different days (D6 to D12, corresponding to cells with increasing maturity). Blood platelets (PLT) were studied as a control for the more mature cells of the lineage. Increase of MYH9 and decrease of MYH10 at mRNA and protein levels were detected by real time RT–PCR (a) and western blotting (b). (a) Real time RT–PCR was normalized to PPIA. (c,d) MYH10 downregulation along the increase in CD41 and CD42 expression. CD41+MKs were derived from cord blood CD34+cells. Cells were sorted according to CD34, CD41 and CD42 expression at day 10 of culture. MYH9 and MYH10 expressions were analysed by western blotting (c) and real-time RT–PCR (d) in CD34+CD41−cells, and/or CD41lowCD42lowand CD41highCD42highMK. Real-time RT–PCR was normalized to HPRT. (e,f) Expression of MYH10 during murine MK differentiation was analysed by real-time RT–PCR (e) and western blotting (f). Lin−cells were purified from mouse fetal liver (Lin-D0, analysed by western blotting) and cultured in the presence of TPO and SCF for 3 days. After 24 h, CD41+cells were sorted from total population (D1, analysed by RT–PCR) and analysed at day 1, 2 and 3 of culture (D1–3 CD41+). (e) Expression of MYH10 transcripts was studied by real-time RT–PCR and normalized to HPRT. (f) Expression of MYH9 and MYH10 proteins by western blots. (g,h) MYH10 localization in human MK derived from CD34+cells from bone marrow. Cells were stained for tubulin (α and β, green) and MYH10 (red). DNA was stained with TOTO (blue). Localization of MYH10 in dipolar 2N–4N mitotic/endomitotic MK (g) and in 4N–8N multipolar endomitosis (h) Scale bars represent 10 μm. (i,j) Comparison of the localization of MYH10 (green) and MYH9 (red) in dipolar mitotic/endomitotic human MK (i) and (j) of dipolar mitotic/endomitotic human MK. DNA was stained with TOTO (blue). Scale bars represent 10 μm. (a,d,e) Error bars represent s.d. of triplicate wells of one experiment. (b,c,f) Anti-HSC70 was used as the control of protein loading. Figure 2: MYH10 is expressed during MK differentiation. ( a , b ) CD41 + MKs were derived from adult blood CD34 + cells and studied at three different days (D6 to D12, corresponding to cells with increasing maturity). Blood platelets (PLT) were studied as a control for the more mature cells of the lineage. Increase of MYH9 and decrease of MYH10 at mRNA and protein levels were detected by real time RT–PCR ( a ) and western blotting ( b ). ( a ) Real time RT–PCR was normalized to PPIA. ( c , d ) MYH10 downregulation along the increase in CD41 and CD42 expression. CD41 + MKs were derived from cord blood CD34 + cells. Cells were sorted according to CD34, CD41 and CD42 expression at day 10 of culture. MYH9 and MYH10 expressions were analysed by western blotting ( c ) and real-time RT–PCR ( d ) in CD34 + CD41 − cells, and/or CD41 low CD42 low and CD41 high CD42 high MK. Real-time RT–PCR was normalized to HPRT. ( e , f ) Expression of MYH10 during murine MK differentiation was analysed by real-time RT–PCR ( e ) and western blotting ( f ). Lin − cells were purified from mouse fetal liver (Lin-D0, analysed by western blotting) and cultured in the presence of TPO and SCF for 3 days. After 24 h, CD41 + cells were sorted from total population (D1, analysed by RT–PCR) and analysed at day 1, 2 and 3 of culture (D1–3 CD41 + ). ( e ) Expression of MYH10 transcripts was studied by real-time RT–PCR and normalized to HPRT. ( f ) Expression of MYH9 and MYH10 proteins by western blots. ( g , h ) MYH10 localization in human MK derived from CD34 + cells from bone marrow. Cells were stained for tubulin (α and β, green) and MYH10 (red). DNA was stained with TOTO (blue). Localization of MYH10 in dipolar 2N–4N mitotic/endomitotic MK ( g ) and in 4N–8N multipolar endomitosis ( h ) Scale bars represent 10 μm. ( i , j ) Comparison of the localization of MYH10 (green) and MYH9 (red) in dipolar mitotic/endomitotic human MK ( i ) and ( j ) of dipolar mitotic/endomitotic human MK. DNA was stained with TOTO (blue). Scale bars represent 10 μm. ( a , d , e ) Error bars represent s.d. of triplicate wells of one experiment. ( b , c , f ) Anti-HSC70 was used as the control of protein loading. Full size image We used immunofluorescence labelling to investigate the recruitment of MYH10 to the contractile ring of mitotic and endomitotic human MK at day 6 of culture. At the 2N–4N transition, MYH10 accumulated at the midzone when the cleavage furrow started to form ( Fig. 2g ), and the percentage of positive cells increased with telophase progression. Only 24.5% of the cells ( n =85, three independent experiments) with a cleavage furrow whose depth remained lower than 75% of cell transversal diameter accumulated MYH10. At later stage, telophase (depth of cleavage furrow >75%), 57% of the cells ( n =141, three independent experiments) showed MYH10 accumulation. In multipolar endomitotic MK (4N to 8N or >8N), only 9% of the cells ( n =42; three independent experiments) with a cleavage furrow lower than 75% of the cell transversal diameter showed MYH10 accumulation and the protein was not located on the whole furrow ( Fig. 2h ). The percentage increased to 29% at the end of telophase (cleavage furrow >75% transversal diameter, 3 independent experiments and 17 late telophase cells counted). Moreover, MYH9 was diffusively present in the cytoplasm of endomitotic MK, whereas MYH10 was specifically localized in the contractile ring (midzone and midbody; Fig. 2i and j ). Only a few human MK accumulated MYH9 at the cleavage furrow at the end of telophase [6] . Furthermore, we found that MYH9 did not accumulate in the contractile ring of dipolar murine MK in telophase (97 telophase cells were counted, 3 independent experiments). These results suggest that MYH10 is the main myosin II isoform present in the contractile ring of MK. Its downregulation during differentiation leads to a decreased myosin II accumulation in the contractile ring. MYH10 is involved in MK ploidy regulation To determine if MYH10 is really implicated in MK polyploidization, human progenitors (CD34 + cells) were induced towards MK differentiation (stem cell factor (SCF)+TPO) and transduced at days 2 and 3 of culture with lentiviruses encoding green fluorescent protein (GFP) and two different short hairpin RNAs (shRNAs) targeting MYH10 (B3 and B5) or a scramble shRNA. Western blot analysis of the GFP-positive population sorted at 72 h after infection with the shMYH10-B5 showed an ~50% reduction in the MYH10 protein level, whereas the level of MYH9 protein remained unchanged ( Fig. 3a ). MYH10 knockdown resulted in a marked increase in MK ploidy, as attested by a shift in mean ploidy from 7.65N to 9.84N for shRNA-treated MK ( n =3, P =0.015, t -test; Fig. 3b ). The shMYH10-B3 was less effective in the downregulation of MYH10 ( Fig. 3a ), as well as in the increase of ploidy. By overexpressing a MYH10 mutated form, not identified by the shRNA, we could confirm in the COS7 cell line that shMYH10 affects the cell cycle by a specific MYH10 knockdown and not by an off-target effect ( Supplementary Fig. S1 ). Conversely, we re-expressed MYH10 in MK at day 5 of culture, using a vector containing MYH10 in fusion with GFP by nucleofection. Quantitative RT–PCR analysis of the GFP-positive populations (MYH10–GFP and control GFP) 48 h after nucleofection showed a 20-fold increase in MYH10 mRNA level, whereas MYH9 mRNA level remained unchanged ( Fig. 3c ). MYH10 overexpression increased the percentage of 2N MK from 30.5 to 41.9% ( n =4, P =0.009, t -test) and reduced MK mean ploidy level (from 6.5N to 5.2N, n =4, P =0.01, t -test; Fig. 3d ). Altogether, these results suggest that MYH10 is the main myosin II isoform implicated in MK polyploidization. 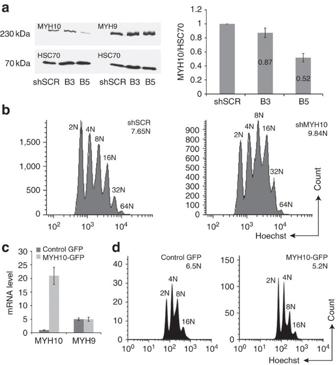Figure 3: Changes in ploidy level induced by MYH10 knockdown or overexpression. (a) Effect of shMYH10 on the level of MYH10 protein in human MK. Protein level was ascertained by western blotting. Anti-HSC70 was used as control of protein loading. (b) MYH10 knockdown increases human MK mean ploidy from 7.65N (shSCR control) to 9.84N (shMYH10 B5). GFP++MK analysed at day 9 of culture (n=3,P=0.015,t-test). (c) Transfection of a plasmid containing MYH10 in fusion with GFP induces overexpression of MYH10 mRNA in MK. Real-time RT–PCR was normalized toHPRT(n=4,P=0.01,t-test, error bars represent s.d. of triplicate wells from one experiment). (d) Overexpression of MYH10 in MK induces an increase in 2N (n=4,P=0.009,t-test) and a decrease in 8N cells (n=4,P=0.01,t-test). Figure 3: Changes in ploidy level induced by MYH10 knockdown or overexpression. ( a ) Effect of shMYH10 on the level of MYH10 protein in human MK. Protein level was ascertained by western blotting. Anti-HSC70 was used as control of protein loading. ( b ) MYH10 knockdown increases human MK mean ploidy from 7.65N (shSCR control) to 9.84N (shMYH10 B5). GFP ++ MK analysed at day 9 of culture ( n =3, P =0.015, t-test ). ( c ) Transfection of a plasmid containing MYH10 in fusion with GFP induces overexpression of MYH10 mRNA in MK. Real-time RT–PCR was normalized to HPRT ( n =4, P =0.01, t -test, error bars represent s.d. of triplicate wells from one experiment). ( d ) Overexpression of MYH10 in MK induces an increase in 2N ( n =4, P =0.009, t -test) and a decrease in 8N cells ( n =4, P =0.01, t -test). Full size image Myosin II is activated during furrow ingression We then investigated if this low myosin accumulation in the contractile ring was capable to generate a myosin activity. Activation of myosin II was assessed by exploring the phosphorylation status of its regulatory light chain (MLC2) with an antibody recognizing PPMLC2-, Ser 19 - and Thr 18 -phosphorylated forms of MLC2. A positive signal was easily seen at late telophase in 68.6% ( n =102, three independent experiments) of dipolar mitotic/endomitotic MK with a cleavage furrow ≥75% cell transversal diameter ( Fig. 4a ). PPMLC2 was also detected on the cleavage furrow of polyploid endomitotic MK examined at late telophase or during cytokinesis failure ( Fig. 4b ), but only for a minority of them (25%, n =24, three independent experiments). This experiment indicates that there still exists some myosin II activity at the contractile ring at the end of MK telophase, even with a reduced myosin heavy chain accumulation. 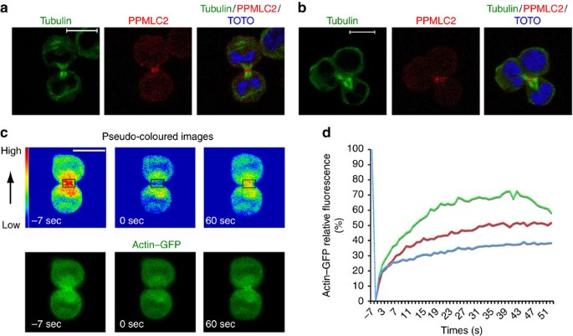Figure 4: Myosin II is in an active state in the contractile ring of MK. (a,b) Human MKs were fixed and stained by an antibody recognizing Ser19- and Thr18-phosphorylated MLC2 (PPMLC2, red) to examine myosin II activation. In both dipolar mitotic/endomitotic MK (a) and multipolar endomitotic MK (b), PPMLC2 was seen at the end of telophase in the midbody. Scale bars represent 10 μm. (c) Contractile ring in late telophase of a dipolar human MK was photobleached and images were acquired every second for 1 min after photobleaching. MKs were transfected with a plasmid encoding a fusion protein between actin and GFP (actin–GFP). The area outlined by the black square is the bleached region. Pseudo-coloured images with rainbow Lut according to GFP-signal intensity and GFP–actin of the corresponding images were presented. Times indicated are before (−7 s) or after (0 s and 60 s) bleaching. Scale bars represent 10 μm. (d) Corresponding graphs of actin–GFP fluorescence recovery in the contractile ring of CD41+MK (red line), CD41−non-MK cells (green line) and MK treated with 12.5 μM blebbistatin (blue line). Figure 4: Myosin II is in an active state in the contractile ring of MK. ( a , b ) Human MKs were fixed and stained by an antibody recognizing Ser 19 - and Thr 18 -phosphorylated MLC2 (PPMLC2, red) to examine myosin II activation. In both dipolar mitotic/endomitotic MK ( a ) and multipolar endomitotic MK ( b ), PPMLC2 was seen at the end of telophase in the midbody. Scale bars represent 10 μm. ( c ) Contractile ring in late telophase of a dipolar human MK was photobleached and images were acquired every second for 1 min after photobleaching. MKs were transfected with a plasmid encoding a fusion protein between actin and GFP (actin–GFP). The area outlined by the black square is the bleached region. Pseudo-coloured images with rainbow Lut according to GFP-signal intensity and GFP–actin of the corresponding images were presented. Times indicated are before (−7 s) or after (0 s and 60 s) bleaching. Scale bars represent 10 μm. ( d ) Corresponding graphs of actin–GFP fluorescence recovery in the contractile ring of CD41 + MK (red line), CD41 − non-MK cells (green line) and MK treated with 12.5 μM blebbistatin (blue line). Full size image MLC2 phosphorylation regulates myosin II activity without affecting the recruitment of myosin II and F-actin in the contractile ring [13] , [17] , [18] and controls the actin dynamics (assembly and disassembly) necessary for completion of cytokinesis [19] . To study actin turnover, CD34 + cells were transfected with a GFP–β-actin construct and induced to differentiate into hematopoietic cells by a cocktail of growth factors. On the basis of the expression of the platelet-specific membrane glycoprotein CD41, GFP-positive cells were sorted into MK (CD41 + GFP + ) and non-MK (CD41 − GFP + ), and actin turnover was measured in the contractile ring at the end of cytokinesis by fluorescence recovery after photobleaching in dipolar mitosis or in endomitosis ( Fig. 4c , Supplementary Movie 1 ). Fluorescence recovery in the contractile ring after bleaching was lower in MK than in non-MK cells (55.7±12.8% with a t 1/2 of 6.3±2.5 s ( n =15) versus 77.6±10.9% with a t 1/2 of 8.6±3.7 s ( n =16); P =0.0007, t -test). This significant decrease in the actin–GFP fluorescence recovery in the contractile ring of MK as compared with control myeloid cells suggested that a high pool of non-dynamic F-actin existed at the end of cytokinesis of dipolar mitotic/endomitotic MK ( Fig. 4d ). Partial inhibition of myosin II activity by blebbistatin pretreatment at low concentration (12.5 μM) increased the fraction of non-dynamic F-actin in the contractile ring of MK, as attested by a decreased fluorescence recovery (42.9±9.0%, with t 1/2 of 2.94±1.35 s, n =8, P =0.01 t -test with blebbistatin; Fig. 4d ). Although blebbistatin is inactivated by blue light, we think that myosin activity was not restored immediately and the time until recovery explains the greater stability of F-actin. Together, these results indicate that a myosin II activity still persists in the contractile ring of MK; however, its attenuation decreased the F-actin mobility, increasing the probability of a cytokinesis failure. To investigate the role of residual myosin II activity on furrow ingression, blebbistatin was added at day 6 of culture when polyploidy begins in MK. Ploidy level was analysed by flow cytometry 72 h later in maturing MK identified by co-expression of two platelet-specific glycoproteins, CD41 and CD42. Blebbistatin significantly increased the mean ploidy from 6.47N to 11.27N at 25 μM ( n =3, P =0.015, t -test; Fig. 5a ) and from 6.28N to 12.12N at 100 μM ( n =4, P =0.008, t -test; Fig. 5b ). When examined by real-time video microscopy, H2B–GFP-expressing MK showed an apparently normal metaphase-to-anaphase transition in the presence of blebbistatin at 25 μM ( Supplementary Movie 2 and 3 ) as compared with controls ( Supplementary Movie 4 and 5 ), but the furrow ingression was almost completely inhibited ( Supplementary Movie 2 and 3 compared with Supplementary Movie 4 and 5 ; Fig. 5c and d ). These data indicated that myosin II was implicated in MK furrow ingression and that its activation had a negative role for MK polyploidization. 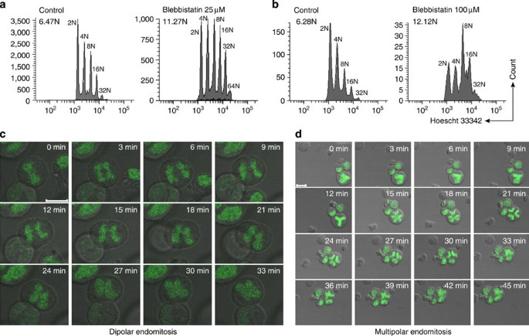Figure 5: Effects of myosin II activity inhibition on MK ploidy and furrow ingression. (a,b) Effects of myosin II inhibitors (blebbistatin) on human MK polyploidization. The ploidy level of CD41+/CD42+MK was analysed at day 9 of culture (72 h after addition of the inhibitor). MK mean ploidy was calculated from the number of cells in each ploidy class (n=3). Blebbistatin was tested at two concentrations: (a) at 25 μM, the mean ploidy level was increased significantly from 6.47N to 11.27N (n=3,P=0.015,t-test), and (b) at 100 μM, from 6.28N to 12.13N (n=4,P=0.008,t-test). (c,d) Human MK transduced with H2B-GFP were treated with blebbistatin (25 μM) and then filmed by real-time video microscopy. Almost no cleavage furrow was seen in diploid (c) and polyploid (d) endomitotic MK. Figure 5: Effects of myosin II activity inhibition on MK ploidy and furrow ingression. ( a , b ) Effects of myosin II inhibitors (blebbistatin) on human MK polyploidization. The ploidy level of CD41 + /CD42 + MK was analysed at day 9 of culture (72 h after addition of the inhibitor). MK mean ploidy was calculated from the number of cells in each ploidy class ( n =3). Blebbistatin was tested at two concentrations: ( a ) at 25 μM, the mean ploidy level was increased significantly from 6.47N to 11.27N ( n =3, P =0.015, t -test), and ( b ) at 100 μM, from 6.28N to 12.13N ( n =4, P =0.008, t -test). ( c , d ) Human MK transduced with H2B-GFP were treated with blebbistatin (25 μM) and then filmed by real-time video microscopy. Almost no cleavage furrow was seen in diploid ( c ) and polyploid ( d ) endomitotic MK. Full size image MYH10 is involved in the switch from mitosis to endomitosis There are two ways to increase MK ploidy: one is to augment the number of endomitotic cycles, the other is to promote the switch from mitosis to endomitosis by preventing 4N cycling cells to return to 2N. To determine the mechanism by which MYH10 knockdown modifies ploidy level, MK cultures were infected at day 0 and day 1 with the shMYH10-B5-encoding lentivirus. The cell cycle status of GFP-positive cells was analysed by bromodeoxyuridine (BrdU) incorporation 72 h after infection (day 4 of culture; three independent experiments). MYH10 knockdown had no effect on BrdU incorporation in both 2N–4N (37% with shMYH10 and 36% with short hairpin scramble sequence (shSCR)) and >4N MK populations (6% with shMYH10 and 8% with shSCR; Fig. 6a ). This result demonstrated that MYH10 knockdown had no impact in the G1/S transition for both diploid and polyploid MK. Simultaneous analysis of the ploidy level showed that MYH10 knockdown diminished the frequency of 2N MK, but increased that of ≥4N MK, suggesting that MYH10 regulates the fate of 4N cells ( Fig. 6b ). To directly demonstrate this mechanism, 4N MKs were sorted after Hoechst 33342 labelling at day 5 of culture and cultured for additional 72 h with and without blebbistatin (25 μM) before ploidy analysis ( Fig. 6c ). After blebbistatin treatment, only a small fraction of 2N MKs were detected (3.4±2.3%), the majority of the cells remained 4N, and a part of MK increased their ploidy level ( Fig. 6c , 4N blebbistatin). Without blebbistatin treatment, a significant fraction of 4N cells returned to 2N, (30±6% 2N MK detected, three independent experiments, P =0.03 t -test; Fig. 6c , 4N control). Collectively, these results demonstrated that MYH10 was involved in the switch from mitosis to endomitosis. This result is in agreement with previous results that have shown that MYH10 is involved in cytokinesis and that its knockdown in cell lines leads to multinucleated polyploid cells [15] , [20] , [21] . 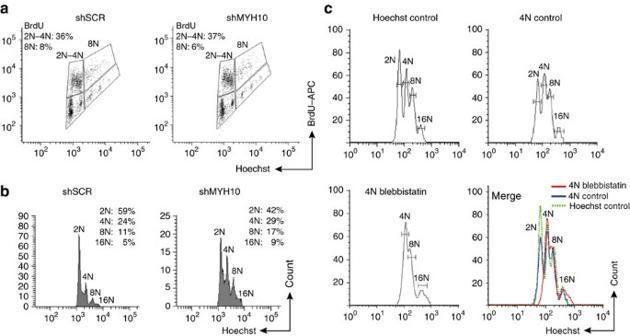Figure 6: Effect of MYH10 knockdown on mitosis to endomitosis transition. (a) BrdU incorporation in the control (shSCR) or after MYH10 knockdown (shMYH10). The BrdU-positive and -negative populations (day 4 of culture) were compared in 2N–4N and >4N MK transduced by shMYH10 (B5) or shSCR control lentivirus. BrdU incorporation in 2N–4N MK was 37% with shMYH10 and 36% with shSCR, and in >4N, MK was 6% with shMYH10 and 8% with shSCR (n=3). (b) Analysis of ploidy levels of GFP+/CD41+MK in the BrdU experiment (day 4 of culture), (c) Effect of blebbistatin on cell cycle of sorted 4N MK. Hoechst control: MKs were incubated with Hoechst 33342 at day 5 of culture for 1 h and cultured for additional 72 h; 4N control: 4N MKs were sorted after Hoechst 33342 labelling at day 5 of culture and cultured for additional 72 h without blebbistatin; 4N blebbistatin: 4N MKs were sorted after Hoechst 33342 labelling at day 5 of culture and cultured for additional 72 h with blebbistatin (25 μM). Merge: Hoechst control, 4N control and 4N blebbistatin. Figure 6: Effect of MYH10 knockdown on mitosis to endomitosis transition. ( a ) BrdU incorporation in the control (shSCR) or after MYH10 knockdown (shMYH10). The BrdU-positive and -negative populations (day 4 of culture) were compared in 2N–4N and >4N MK transduced by shMYH10 (B5) or shSCR control lentivirus. BrdU incorporation in 2N–4N MK was 37% with shMYH10 and 36% with shSCR, and in >4N, MK was 6% with shMYH10 and 8% with shSCR ( n =3). ( b ) Analysis of ploidy levels of GFP + /CD41 + MK in the BrdU experiment (day 4 of culture), ( c ) Effect of blebbistatin on cell cycle of sorted 4N MK. Hoechst control: MKs were incubated with Hoechst 33342 at day 5 of culture for 1 h and cultured for additional 72 h; 4N control: 4N MKs were sorted after Hoechst 33342 labelling at day 5 of culture and cultured for additional 72 h without blebbistatin; 4N blebbistatin: 4N MKs were sorted after Hoechst 33342 labelling at day 5 of culture and cultured for additional 72 h with blebbistatin (25 μM). Merge: Hoechst control, 4N control and 4N blebbistatin. Full size image RUNX1 mediates MYH10 silencing during MK differentiation The arrest of endomitosis is linked to MK maturation and RUNX1 has a role in this process by regulating genes involved in platelet functions, including myosin light chain 9 (MYL9/MLC2 ) [22] and the CDK inhibitor p19 INK4D (ref. 23 ). Small diploid MKs are present in the bone marrow of runx1 KO mice [24] , [25] suggesting that RUNX1 could also regulate the switch from mitosis to endomitosis by targeting MYH10. Using an in silico approach with the ChipMapper online software, we identified a putative conserved RUNX1 transcription factor-binding site in the MYH10 promoter region ( Fig. 7a , Supplementary Fig. S2 ). Chromatin immunoprecipitation (ChIP) assays demonstrated that RUNX1 could bind this site in MK ( Fig. 7b , two independent experiments were performed). To test for its functional relevance, we cloned the promoter region (pMYH10_luc) with or without mutation in the RUNX1-binding site (pMYH10mut_luc) upstream of the luciferase gene ( Fig. 7a ). We performed gene reporter assays in the human erythroleukemia cell line. The mutation in the RUNX1-binding site led to a significant increase in luciferase activity ( n =3, P ≤0.05, t -test; Fig. 7c ). To better understand the regulatory role of RUNX1 in MK, we then transduced human CD34 + cells induced for MK differentiation at day 1 and day 2 of culture with a lentivirus encoding an shRNA-targeting RUNX1 (shRUNX1) [23] . As shown in Fig. 7d , shRUNX1 treatment led to a significant decrease (30–50% depending on experiment) in the RUNX1 transcripts. Real-time PCR showed a 1.5-fold increase in MYH10 expression ( Fig. 7d ), which was confirmed at the protein level ( Fig. 8a ), whereas flow cytometric analysis showed a decrease in the ploidy level of mature MK (CD41 high CD42 high ; n =3, P ≤0.01, t -test; Fig. 8b ). 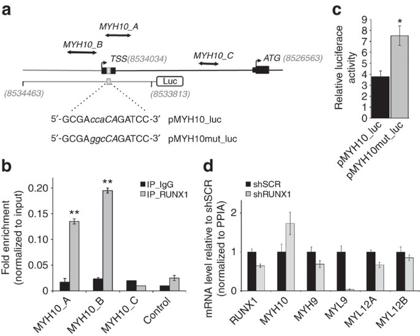Figure 7: RUNX1 regulates negatively MYH10 transcription during MK differentiation. (a) Schematic representation of MYH10 promoter. Gray numbers indicate genomic location in the UCSC database (GRCh37/hg19). Gray box indicates RUNX1 putative binding site and black lines show MYH10_A, _B, and _C amplicon fragments studied in ChIP experiment, respectively, localized in position: chr17:8533904–8534036, chr17:8534067–8534201, chr17:8530973–8531054. TSS indicates transcription start site. (b) Quantitative ChIP analysis was performed in MK. Primers encompassing (MYH10_Aand_B) or not (MYH10_C)the RUNX1 site were used to amplify input genomic DNA, and the DNA precipitated by antibodies against either normal immunoglobulin G (IgG) or RUNX1. A genomic region without RUNX1-binding site was used as negative control sequence (control). Values are normalized to input genomic DNA. Values obtained for fold enrichment using MYH10_A and B were statistically significant as indicated. All the data are representative of three independent experiments performed in duplicate (n=3, **P≤0.01,t-test, error bars represent s.d. of duplicate). (c) MYH10-promoter luciferase assay with (pMYH10mut_luc) or without mutated RUNX1-binding site (pMYH10_luc) in human erythroleukemia (HEL) cells. Two independent experiments were performed. (c) Illustrates one representative experiment (n=3, *P≤0.05 error bars represent s.d.). (d) CD41+CD42+GFP+cells were sorted at day 6 of culture in presence of TPO. RUNX1, MYH10, MYH9, MYL9, MYL12A and MYL12B expression levels were analysed by real-time RT–PCR, expression level was normalized to PPIA and expressed relatively to shSCR (control). Error bars represent s.d. of triplicate wells from one experiment. Figure 7: RUNX1 regulates negatively MYH10 transcription during MK differentiation. ( a ) Schematic representation of MYH10 promoter. Gray numbers indicate genomic location in the UCSC database (GRCh37/hg19). Gray box indicates RUNX1 putative binding site and black lines show MYH10_A, _B, and _C amplicon fragments studied in ChIP experiment, respectively, localized in position: chr17:8533904–8534036, chr17:8534067–8534201, chr17:8530973–8531054. TSS indicates transcription start site. ( b ) Quantitative ChIP analysis was performed in MK. Primers encompassing ( MYH10_A and _B ) or not ( MYH10_C) the RUNX1 site were used to amplify input genomic DNA, and the DNA precipitated by antibodies against either normal immunoglobulin G (IgG) or RUNX1. A genomic region without RUNX1-binding site was used as negative control sequence (control). Values are normalized to input genomic DNA. Values obtained for fold enrichment using MYH10_A and B were statistically significant as indicated. All the data are representative of three independent experiments performed in duplicate ( n =3, ** P≤ 0.01, t -test, error bars represent s.d. of duplicate). ( c ) MYH10-promoter luciferase assay with (pMYH10mut_luc) or without mutated RUNX1-binding site (pMYH10_luc) in human erythroleukemia (HEL) cells. Two independent experiments were performed. ( c ) Illustrates one representative experiment ( n =3, * P≤ 0.05 error bars represent s.d.). ( d ) CD41 + CD42 + GFP + cells were sorted at day 6 of culture in presence of TPO. RUNX1, MYH10, MYH9, MYL9, MYL12A and MYL12B expression levels were analysed by real-time RT–PCR, expression level was normalized to PPIA and expressed relatively to shSCR (control). Error bars represent s.d. of triplicate wells from one experiment. 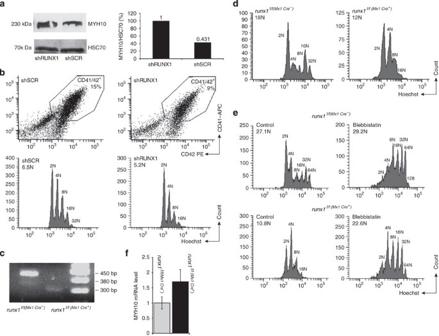Figure 8: Effects of RUNX1 knockdown or KO on MYH10 expression and MK ploidy level in human and mouse. (a) shRNA-mediated RUNX1 knockdown increases MYH10 protein level (western blots) in sorted GFP+human MK at day 9 of culture. (b) At day 9 of culture, ploidy levels were analysed by flow cytometry in CD41+CD42+GFP+human cells (n=3,P≤0.01,t-test). shRNA-mediated RUNX1 knockdown decreases MK ploidy level. (c) Five weeks after induction ofrunx1KO by injection of pIpC, the excision by Cre-recombinase ofrunx1locus flanked by LoxP sites was verified by PCR on DNA isolated from bone marrow progenitors (Lin−cells). (d) The effect ofrunx1KO on ploidy level was analysed directly on bone marrow murine CD41+MK. (e) At day 2.5 in culture, ploidy level in MK derived fromrunx1f/f(Mx1 Cre+)mouse bone marrow was analysed by flow cytometry in CD41+cells cultured with (50 μM) or without blebbistatin (forrunx1f/f(Mx1 Cre+)mice,n=3,P=0.006,t-test; forrunx1f/f(Mx1 Cre-)mice,n=4,P=0.02,t-test). (f) At day 2.5 in culture, CD41+cells derived fromrunx1f/f(Mx1 Cre+)mouse bone marrow were sorted and MYH10 expression level was analysed. Real-time RT–PCR was normalized to HPRT (a pool of CD41+cells from threerunx1f/f(Mx1 Cre+)mice and from fourrunx1f/f(Mx1 Cre-)mice was analysed). Error bars represent s.d. of triplicate. Full size image Figure 8: Effects of RUNX1 knockdown or KO on MYH10 expression and MK ploidy level in human and mouse. ( a ) shRNA-mediated RUNX1 knockdown increases MYH10 protein level (western blots) in sorted GFP + human MK at day 9 of culture. ( b ) At day 9 of culture, ploidy levels were analysed by flow cytometry in CD41 + CD42 + GFP + human cells ( n =3, P ≤0.01, t -test). shRNA-mediated RUNX1 knockdown decreases MK ploidy level. ( c ) Five weeks after induction of runx1 KO by injection of pIpC, the excision by Cre-recombinase of runx1 locus flanked by LoxP sites was verified by PCR on DNA isolated from bone marrow progenitors (Lin − cells). ( d ) The effect of runx1 KO on ploidy level was analysed directly on bone marrow murine CD41 + MK. ( e ) At day 2.5 in culture, ploidy level in MK derived from runx1 f/f(Mx1 Cre+) mouse bone marrow was analysed by flow cytometry in CD41 + cells cultured with (50 μM) or without blebbistatin (for runx1 f/f(Mx1 Cre+) mice, n =3, P =0.006, t -test; for runx1 f/f(Mx1 Cre-) mice, n =4, P =0.02, t -test). ( f ) At day 2.5 in culture, CD41 + cells derived from runx1 f/f(Mx1 Cre+) mouse bone marrow were sorted and MYH10 expression level was analysed. Real-time RT–PCR was normalized to HPRT (a pool of CD41 + cells from three runx1 f/f(Mx1 Cre+) mice and from four runx1 f/f(Mx1 Cre-) mice was analysed). Error bars represent s.d. of triplicate. Full size image To confirm these results in vivo , we used a KO mouse model in which the conditional runx1 f/f mouse strain [24] was crossed with Mx1-Cre mice. Efficient Runx1 deletion was achieved in hematopoietic cells depleted in lineage markers (lineage-negative (Lin − )) 5 weeks after injection of polyinosinic-polyacytidylic acid (pIpC) ( Fig. 8c ) [24] . Runx1 -deficient bone marrow MK exhibited a decrease in ploidy level, as compared with control littermates (mean ploidy 12N versus 18N; n =3, P ≤0.01, t -test; Fig. 8d ). Bone marrow Lin − cells were cultured in the presence of TPO, and CD41 + cells were sorted at day 2.5 of culture. Blebbistatin (50 μM) induced a dramatic increase in ploidy in runx1 f/f(Mx1 Cre+) MK (mean ploidy from 10.8N to 22.6N, n =3, P =0.006, t -test; Fig. 8e ). A significant 1.7-fold increase of Myh10 mRNA level was detected in runx1 -deficient MK ( Fig. 8f ). Altogether, the RUNX1/MYH10 pathway appears as an important regulator of the switch from mitosis to endomitosis. The mechanism of the switch from mitosis to endomitosis in MK is still a matter of controversy [26] , [27] , [28] , [29] , [30] with studies suggesting a cell cycle regulation defect, whereas others argue for a defect in the expression of the central spindle proteins. Our new findings demonstrate the key contribution of MYH10 downregulation in the process of the switch from mitosis to endomitosis. Evidence was provided that endomitosis was a defect in late cytokinesis with an incomplete furrow ingression [5] , [6] , [7] . Here we demonstrate that immature MK express myosin IIB and that the MYH10 gene is silenced during differentiation. We also show that the two non-muscle myosin II isoforms have distinct roles in MK. By accumulating in the contractile ring, MYH10 is involved in late phases of mitosis, whereas MYH9 appears to be mainly an organizer of the MK cytoplasm and is implicated in pro-platelet formation at late stages of differentiation [10] , [12] . Sustaining this hypothesis, a limited MYH9 accumulation was observed in the contractile ring of human MK [6] . Furthermore, MYH9 was not detected in the cleavage furrow of murine MK and an myh9 KO did not modify the MK ploidy [12] . Therefore, it is likely that non-muscle myosin IIA and B have two distinct functions, both in human and murine megakaryopoiesis. These two myosin II isoforms have previously been shown to have distinct roles in cadherin junction of the epithelial cells [31] or in the erythroblast enucleation [32] . However, MYH10 silencing does not explain the entire polyploidization process. MYH10 silencing has a central role at the 2N–4N transition in MK by inducing failure of cytokinesis as also observed in MYH10-ablated cardiac myocytes [21] or COS cells [15] , [20] . However, MKs are not subsequently blocked in 4N. Thus, abnormalities in the G1/S transition check point might also be present in the 4N MK [3] , [33] , [34] . In addition, it remains to understand why MYH9 does not accumulate in the cleavage furrow of MK in contrast to other cell types; in fact, myosin II isoform localization may depend on distinct upstream signalling pathways as shown in epithelial cells [31] . RUNX1, one of the main transcription factor involved in MK differentiation, directly regulates MYH10 expression and is responsible for its repression during MK differentiation, which may explain the presence of low ploidy MK in runx1 f/f(Mx1 Cre+) mice [24] , [25] , as well as in hereditary or acquired haematological disorders associated with RUNX1 loss-of-function mutations [35] , [36] . Low-ploidy MK has been observed in KO of other transcription factors, such as GATA1 or FLI-1 (refs 37 , 38 ). As these two transcription factors may be associated with RUNX1 in large transcription complexes [39] , [40] , they may similarly act on MYH10 expression. The observation that two non-muscle myosin II isoforms are present in MK and have distinct roles opens new avenues of research; for example, the MYH9/MYH10 ratio could be used as a marker of MK differentiation and dysfunction. Complete understanding of how MYH10 expression is regulated in numerous physiological and pathological conditions remains a question for further investigations. Mice and in vitro cultures of murine MK The conditional runx1 KO mouse strain was developed by Dr J. D. Growney et al . [24] and was a gift from Dr. D. G. Gilliland (Boston, USA) and Dr. N. A. Speck (Philadelphia, USA). Runx1 f/f mice were crossed with Mx1-Cre mice; deletion of runx1 locus flanked by LoxP sites was induced by injection of the interferon-inducing agent pIpC. Five weeks after runx1 KO induction, platelet counts were performed. The runx1 KO mice exhibited thrombopenia (2–3×10 5 platelets per ml), contrasting with mice negative for Cre-recombinase (~1×10 6 platelets per ml). The floxed myh9 strain was crossed with PF4-Cre mice to obtain mice with deletion of the MYH9 exon 1 in the MK lineage, as described previously [11] . Lin − cells were purified from the fetal liver (E14.5) after incubation with a mixture of rat monoclonal antibodies against lineage antigens (Gr1, TER119, CD11b, B220 and anti-CD3, 15 μg ml −1 each, Pharmingen, CA, USA) and depleted with Dynabeads coupled to a mouse antibody against rat immunoglobulin (Dynal, Norway). Lin − cells were cultured in the presence of murine (SCF, 10 ng ml −1 , Peprotech, USA) and TPO (50 ng ml −1 , Kirin Brewery, Tokyo, Japan) to obtain murine MK. Blebbistatin (50 μM) was added at the onset of Lin − cell culture and MK ploidy was analysed after 48 h treatment by blebbistatin. Mice were housed and analysed at the Institut Gustave Roussy Animal Facilities (Villejuif, France) according to the national and institutional guidelines. In vitro MK culture derived from human CD34 + cells CD34 + cells were obtained in agreement with our Institute Ethic Committee (Assistance Publique des Hôpitaux de Paris) from the bone marrow of healthy patients, leukapheresis samples and cord blood. CD34 + cells were isolated by an immunomagnetic cell sorting technique (AutoMacs; Miltenyi Biotec, Germany) and cultured in serum-free medium in the presence of recombinant human TPO (10 ng ml −1 ) [41] . Depending on the experiments, MKs were sorted according to CD41, or CD41 and CD42 expression using Influx flow cytometer (BD, Mountain View, CA) [42] . Fluorescence recovery after photobleaching analysis CD34 + cells were cultured 4 days in serum-free medium with recombinant human cytokines: either a combination of TPO (10 ng ml −1 ) and SCF (25 ng ml −1 ; Biovitrum AB, Stockholm, Sweden) or a combination of TPO, interleukin-3 (100 U ml −1 , Novartis, Basle, Switzerland), SCF and fetal liver tyrosine kinase ligand (10 ng ml −1 , Celldex Therapeutics Inc., Needham, USA). Cells were then transfected with the GFP–β-actin construct by the Amaxa nucleofection system (Amaxa, France). Twenty-four hours after transfection, CD41 + GFP + MKs were sorted. The CD41 − GFP + cells (mainly myeloid precursors) were obtained from cultures performed with four growth factors and were used as control. Hoechst 33342 (5 μg ml −1 , Sigma, France) was added in the medium 5 min before observation under a laser-scanning microscope (LSM). In some experiments, blebbistatin, an enantiomer mixture of blebbistatin (±), (Merck, Germany) disolved in dimethyl sulfoxide (DMSO; 12.5 μM) or the same volume of diluents (DMSO) was added in the medium 30 min before observation. Photobleaching experiments were performed with a Zeiss LSM (510, Carl Zeiss, Germany) using a ×63/1.4 numerical aperture oil objective at 37 °C with 5% CO 2 in air. Bleaching of the marked region was carried out at 100% laser power with 100 iterations. After photobleaching, images were acquired every second for 1 min. Fluorescence recovery was analysed with the Zeiss Image Examiner and Excel softwares. Lentiviral constructs The EF1α-H2BGFP fragment from the BOS-H2BGFP vector (BD Pharmingen) was excised and subcloned into an HIV-derived lentiviral vector (pRRLsin-PGK-eGFP-WPRE; Genethon, France) in place of the phosphoglycerate kinase (PGK)-enhanced GFP sequence. shRNA cloning and lentiviral construction shRUNX1-containing lentivirus was previously described [23] . Two shMYH10, and control SCR containing lentiviruses were constructed as previously described [23] . Lentivirus production Lentivirus particles were prepared by transient co-transfection of human HEK293T cells with lentiviral vector plasmids (H2B-GFP [6] , shRNA MYH10, shRNA RUNX1, shRNA SCR), the packaging plasmid pCMVΔR8.74 and the VSV-G protein envelope plasmid. JetPrime (Ozyme, France) was used for transfection according to the manufacturer's instructions. Lentivirus stocks containing about 10 9 infectious particles per ml were kept frozen at −70 °C. Viruses stocks were thawed and immediately used. Cell transduction CD34 + cells were cultured with TPO and SCF. Lentiviral particles were added at a concentration of 10 7 infectious particles per 1×10 5 cells for 12 h followed by a second transduction, then cells were cultured in presence of TPO [23] . Electroporation pEGFP-C3-MHCB plasmid encoding for wild-type MYH10 cDNA was kindly provided by Professor Shoshana Ravid (The Hebrew University, Israel). To test for specificity of the shMYH10 in COS7 cell line, four nucleotides localized in the region recognized by the shMYH10 were mutated in MYH10 cDNA by directed mutagenesis (3928nt gcagc T / A ag T / C cttgagtc T / C ca A / G 3949nt, NM_005964.1). To study MYH10 overexpression in primary MK, the cytomegalovirus promoter was replaced by the EF1α promoter. pEGFP-EF1α-MHCB and the control (pEGFP-EF1α) were delivered into MK by nucleofection (Amaxa Inc., MD). BrdU analysis CD34 + cells were cultured with TPO and SCF, and transduced by the shMYH10 or shSCR at day 0 and day 1 culture. GFP + cells sorted at day 4 of culture were incubated with 10 μM BrdU for 1 h at 37 °C. Staining was performed with the BrdU flow kit according to manufacturer's instruction (BD Pharmingen). BrdU incorporation was analysed in CD41 + cells stained with propidium iodide on a LSRII (Becton Dickinson). Ploidy analysis Hoechst 33342 (10 μg ml −1 ) was added in the medium of cultured MK for 1 h at 37 °C. Cells were stained with directly coupled monoclonal antibodies: anti-CD41 APC and anti-CD42 PE (BD Biosciences) for 30 min at 4 °C [26] . Ploidy was measured in the CD41 + /CD42 + cell population (for chemical inhibitors test) and in the CD41 + /CD42 + /GFP + population (after lentiviral transduction) by means of a LSRII flow cytometer equipped with three lasers (360, 480 and 560 nM excitation; Becton Dickinson). The mean ploidy of human MK was calculated by the following formula: (2N×the number of cells at 2N ploidy level +...+64N×the number of cells at 64N ploidy level/the total number of cells). The mean ploidy of murine MK was calculated in ≥8N MK. Mitosis and endomitosis transition analysis Hoechst 33342 (4 μg ml −1 ) was added in the medium for 1 h at 37 °C before cell sorting at day 5 of culture. The 4N sorted cells were cultured for additional 72 h with and without blebbistatin (25 μM) before ploidy analysis in the CD41 + population described above. Western blot analysis Cells were lysed in Laemmli 2× buffer, and the lysates were then gently sonicated on ice. Samples were boiled 5 min in loading buffer and subjected to SDS–polyacylamide gel electroporesis gel. After transfer, nitrocellulose membranes were blotted with the following antibodies: rabbit anti-MYH10, anti-MYH9 (Cell Signaling, Cat. Number 3404 and Number 3403, both diluted at 1:1000) and anti-HSC70 antibodies (Stressgen, used at 0.2 μg ml −1 ) followed by horseradish peroxidase-linked secondary antibodies and Immobilon Western Chemiluminescent HRP Substrate (Millipore Corporation, USA). Immunofluorescence Immunofluorescence was performed on CD41 + MK sorted at day 6 of human culture [42] or day 2 of murine culture derived from Lin − liver fetal cells. Cells were examined under the Zeiss LSM. The following antibodies were used: rabbit anti-MYH10 and anti-MYH9 antibodies (as above, both diluted at 1:100), mouse anti-MYH9 (Sigma, used at 10 μg ml −1 ), rabbit anti-phospho-MLC2 Thr 18 Ser 19 (PPMLC2; gift from Dr J. M. Staddon) [43] , and mouse anti-α tubulin and anti-β tubulin antibodies (Sigma, both used at 20 μg ml −1 ). Appropriate secondary antibodies were conjugated with Alexa 488 or Alexa 546 (Molecular Probes). TOTO-3 iodide (Molecular Probes) was applied for nucleus staining. Live-cell imaging by confocal video microscopy CD34 + cells were cultured 3 days in the presence of TPO and then transduced by H2B-GFP lentivirus as previously described [6] . After transduction, cells were cultured in the presence of TPO for 48–72 h. Cells were then seeded in glass bottom culture dish (MatTek) and were imaged under the Zeiss LSM using a ×63/1.4 numerical aperture oil objective at 37 °C with 5% CO 2 in air. Serial images were obtained at 3- or 5-min interval. Image analyses were performed with the Zeiss Image Examiner software. Quantitative real-time PCR The mRNA isolation, reverse-transcription, and RT–PCR analyses were performed as described [23] . The expression levels of all genes studied were expressed relatively to housekeeping genes, PPIA for human cells and HPRT for murine cells, where the PPIA level was not comparable to that of MYH10. Primer sequences are listed in Supplementary Table S1 . ChIP and promoter activity assays ChIP assays were performed with a ChIP assay kit (Millipore Upstate Biotechnology) using the anti-RUNX1 antibody (8 μg per sample, sc-65, Santa Cruz Biotechnology). Assays were performed using chromatin prepared from human MK as previously described [23] . Immunoprecipitated DNA was analysed on a PRISM ® 7700 sequence detection system using SYBR ® green (Applied biosystems) in duplicate. Primer sequences are listed in Supplementary Table S1 . Luciferase reporter assay The human erythroleukemia cells were transfected with the reporter plasmids, pMYH10_luc and pMYH10mut_luc, and co-transfected with TK-Renilla reporter (Promega, France) for normalization of transfection efficiency. Transfected cells were harvested at 48 h post-transfection. A dual luciferase assay was performed according to the manufacturer′s instructions (Promega, France). The luciferase activity was measured with an AutoLumat LB953 luminometer (Berthold). Statistics Statistical significance was determined by Student's t -test. A P -value <0.05 was considered as statistically significant. Error bars represent s.d. of duplicate or triplicate. How to cite this article: Lordier, L. et al . RUNX1-induced silencing of non-muscle myosin heavy chain IIB contributes to megakaryocyte polyploidization. Nat. Commun. 3:717 doi: 10.1038/ncomms1704 (2012).